Insights into mitochondrial fatty acid synthesis from the structure of heterotetrameric 3-ketoacyl-ACP reductase/3R-hydroxyacyl-CoA dehydrogenase Mitochondrial fatty acid synthesis (mtFAS) is essential for respiratory growth in yeast and mammalian embryonic survival. The human 3-ketoacyl-acyl carrier protein (ACP) reductase (KAR) of mtFAS is a heterotetrameric α 2 β 2 -assembly composed of 17β-hydroxysteroid dehydrogenase type-8 (HSD17B8, α-subunit) and carbonyl reductase type-4 (CBR4, β-subunit). Here we provide a structural explanation for the stability of the heterotetramer from the crystal structure with NAD + and NADP + bound to the HSD17B8 and CBR4 subunits, respectively, and show that the catalytic activity of the NADPH- and ACP-dependent CBR4 subunit is crucial for a functional Hs KAR. Therefore, mtFAS is NADPH- and ACP dependent, employing the 3R-hydroxyacyl-ACP intermediate. HSD17B8 assists in the formation of the competent Hs KAR assembly. The intrinsic NAD + - and CoA-dependent activity of the HSD17B8 subunit on the 3R-hydroxyacyl-CoA intermediates may indicate a role for this subunit in routing 3R-hydroxyacyl-CoA esters, potentially arising from the metabolism of unsaturated fatty acids, into the mitochondrial β-oxidation pathway. Mitochondria play a crucial role in cellular activities of all eukaryotes, including energy conversion [1] , lipid metabolism [2] , apoptosis [3] and innate immune responses [4] . A new pathway, mitochondrial fatty acid synthesis (mtFAS), has recently gained attention since its physiological significance was recognized [5] . mtFAS is similar to the bacterial FAS-II system, where each of the four catalytic steps are catalysed by distinct enzymes ( Fig. 1 ), while the cytosolic FAS in eukaryotes is carried out by the FAS-I multifunctional enzyme complex. mtFAS provides the precursor of mitochondrially synthesized α-lipoic acid, a key cofactor for oxidative decarboxylation of α-keto acids and glycine within eukaryotic cells [5] . There is evidence for other physiologically relevant products of mtFAS in yeast [6] . Deficiency of mtFAS leads to respiratory chain defects and mitochondrial dysfunction [6] , [7] , [8] . 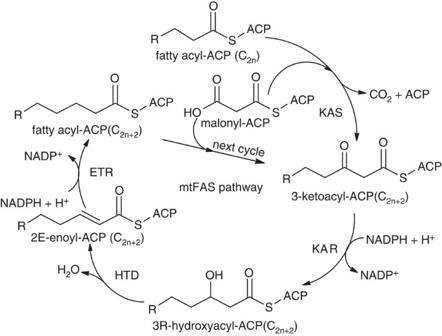Figure 1: Scheme of the human mtFAS pathway showing the mechanism of fatty acyl chain elongation by two carbon units per cycle. The four reactions correspond to KAS (3-ketoacyl-thioester synthase), KAR (3-ketoacyl-thioester reductase), HTD (3-hydroxyacyl-thioester dehydratase) and ETR (2-enoyl-thioester reductase). In our present studies, we show that the KAR activity of the mtFAS pathway is NADPH-dependent as also observed for ETR. Figure 1: Scheme of the human mtFAS pathway showing the mechanism of fatty acyl chain elongation by two carbon units per cycle. The four reactions correspond to KAS (3-ketoacyl-thioester synthase), KAR (3-ketoacyl-thioester reductase), HTD (3-hydroxyacyl-thioester dehydratase) and ETR (2-enoyl-thioester reductase). In our present studies, we show that the KAR activity of the mtFAS pathway is NADPH-dependent as also observed for ETR. Full size image 3-Ketoacyl-acyl carrier protein (ACP) reductase (KAR) catalyses the second step of the mtFAS pathway ( Fig. 1 ). Although all the other mtFAS enzymes identified thus far are encoded by single genes, human KAR ( Hs KAR) is a heterotetrametric α 2 β 2 enzyme formed by two subunits, 17β-hydroxysteroid dehydrogenase type 8 (HSD17B8 or KE6, α-subunit) and carbonyl reductase type 4 (CBR4 or SDR45C1, β-subunit) [9] . Hs HSD17B8 is expressed in abundance in the prostate, placenta and kidney, and has been shown to catalyse the reversible oxidation/reduction of steroid molecules in vitro [10] . The physiological roles of HSD17B8 and CBR4 have remained elusive, and information is only available from studies of the respective homotetramers. The two subunits of Hs KAR belong to the short-chain dehydrogenase/reductase (SDR) superfamily [11] and share 35% sequence identity. However, the orthologues of Hs KAR (fabG or Oar1) studied thus far are homotetrameric. A crystal structure of the Hs HSD17B8 homotetramer is available in the protein data bank (PDB id: 2PD6). Hs CBR4, the other component of Hs KAR, is much less studied and there is no structural information. A previous report shows that CBR4 has quinone reductase activity in vitro [12] . Hs CBR4 displays the highest expression in neuronal and muscle tissues ( http://cgap.nci.nih.gov/ ). It is important to note that when these two proteins are co-expressed in Escherichia coli , they exclusively form α 2 β 2 tetramers rather than forming homotetramers [9] . The heterotetrameric structure triggers the questions why two different subunits are required and what are the roles of the HSD17B8 and the CBR4 subunits in the assembly, substrate recognition and catalysis. The crystal structure of Hs KAR shows that the HSD17B8 and CBR4 subunits complement each other, making a much more stable quaternary structure than the respective homotetramers. Through crystallographic binding studies, structure-guided site-directed mutagenesis, enzyme assays, surface plasmon resonance (SPR) binding studies and in vivo complementation experiments in yeast, we demonstrate that the CBR4 subunit is the functional unit of Hs KAR in mtFAS responsible for NADPH and acyl-ACP binding and catalysis. Thus, this work has identified the biological enzyme function of CBR4. The HSD17B8 subunit works as a scaffold protein, facilitating a competent and functional Hs KAR assembly. In addition, we speculate that this subunit may act as an auxiliary mitochondrial β-oxidation enzyme oxidizing the 3R-hydroxyacyl-CoA metabolites arising from the metabolism of unsaturated fatty acids. Crystal structure of the heterotetrameric Hs KAR Our previous research indicated that Hs KAR is composed of two components, Hs HSD17B8 and Hs CBR4. The crystals of Hs KAR, cocrystallized with NAD + (referred to as Hs KAR-NAD + ), belong to space group P2 1 and diffract up to a resolution of 2.85 Å ( Table 1 ). The crystals contain four tetramers in the asymmetric unit and exhibit pseudomerohedral twinning, with the twin law l, -k, h and twin fraction of ~0.3. The Hs KAR crystal complexed with both NAD + and NADP + (referred to as Hs KAR-NAD(P) + ) was isomorphous to the Hs KAR-NAD + crystals and diffracted up to a resolution of 2.34 Å ( Table 1 ). The pseudomerohedral twinning was almost non-existent in this crystal (0.1). Table 1 Data collection and refinement statistics of Hs KAR. Full size table The tertiary structures of the HSD17B8 and CBR4 subunits are well conserved [13] , [14] , [15] , [16] , [17] , [18] , [19] , [20] ( Fig. 2a ). The general structure of a CBR4 or HSD17B8 monomer features a central parallel β-sheet composed of seven β-strands (β1–β7) sandwiched between helices α1, α2 and α6 on one side and helices α3, α4 and α5 on the other side. Helices α' and α'' are above the strands β6 and β7 ( Fig. 2a ). 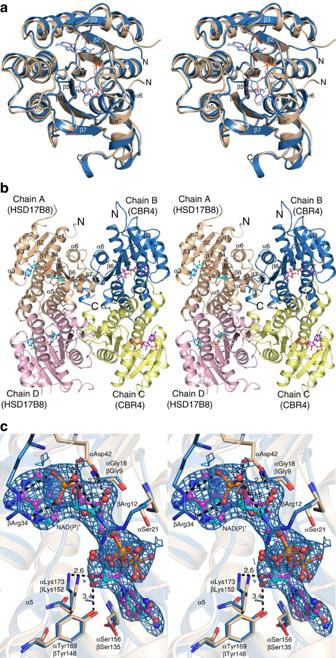Figure 2: Structure ofHsKAR. (a) Cartoon stereo diagram of the monomeric structure ofHsKAR subunits HSD17B8 (α) (brown) and CBR4 (β) (blue). The secondary structure elements are labelled. The N- and C-termini of the polypeptides are marked. (b) The tetrameric organization ofHsKAR in stereo. The two HSD17B8 subunits are represented in brown (chain A) and pink (chain D) cartoon. The two CBR4 subunits are shown in blue (chain B) and yellow (chain C) cartoon. NAD+bound in the two HSD17B8 subunits is represented in cyan ball and stick model (in chain A and D). The two NADP+molecules as bound in the two CBR4 subunits are highlighted in magenta (in chain B and C) ball and stick model. The secondary structure elements are labelled in chain A and selected secondary structure elements are labelled in chain B. (c) Ball and stick model of NAD+(cyan) and NADP+(magenta) as bound to the HSD17B8 and CBR4 subunits, respectively. The HSD17B8 and CBR4 subunits are superimposed to highlight the similar mode of cofactor binding. The residues chosen for mutagenesis on HSD17B8 (brown) and CBR4 (blue) near the cofactor binding site are shown as a ball and stick model. The important interactions are highlighted by black dashes and the distances are shown in angstrom. Superimposed is also the (2Fo–Fc) electron density map of the NADP+contoured at 1σ. Figure 2: Structure of Hs KAR. ( a ) Cartoon stereo diagram of the monomeric structure of Hs KAR subunits HSD17B8 (α) (brown) and CBR4 (β) (blue). The secondary structure elements are labelled. The N- and C-termini of the polypeptides are marked. ( b ) The tetrameric organization of Hs KAR in stereo. The two HSD17B8 subunits are represented in brown (chain A) and pink (chain D) cartoon. The two CBR4 subunits are shown in blue (chain B) and yellow (chain C) cartoon. NAD + bound in the two HSD17B8 subunits is represented in cyan ball and stick model (in chain A and D). The two NADP + molecules as bound in the two CBR4 subunits are highlighted in magenta (in chain B and C) ball and stick model. The secondary structure elements are labelled in chain A and selected secondary structure elements are labelled in chain B. ( c ) Ball and stick model of NAD + (cyan) and NADP + (magenta) as bound to the HSD17B8 and CBR4 subunits, respectively. The HSD17B8 and CBR4 subunits are superimposed to highlight the similar mode of cofactor binding. The residues chosen for mutagenesis on HSD17B8 (brown) and CBR4 (blue) near the cofactor binding site are shown as a ball and stick model. The important interactions are highlighted by black dashes and the distances are shown in angstrom. Superimposed is also the (2 F o – F c ) electron density map of the NADP + contoured at 1 σ . Full size image In the Hs KAR-NAD + structure, the electron density is well defined for the two HSD17B8 subunits (chains A and D) with breaks mainly in the loop region connecting α2 and β3 (residues 56–67), which is slightly longer ( Supplementary Fig. 1 ) compared with the previously studied KARs and Hs CBR4. The electron densities for the CBR4 subunits (chains B and C) are less well defined. Despite slightly better definition of chain B, density for residues 184–194, corresponding to two helices (α' and α''), above the proposed cofactor binding site, is missing. In chain C, residues 39 to 51 comprising helix α2 and part of strand β3 are poorly defined. In chains B and C, many side-chain densities of the surface residues are poor. In the Hs KAR-NAD(P) + structure, the overall electron density is of high quality, also for the CBR4 subunits. In two CBR4 subunits (chains F and J), continuous electron density is present for the entire chain. Owing to its superior diffraction quality and the presence of both the cofactors, the Hs KAR-NAD(P) + structure has been used for the further analysis and comparisons. In each tetramer, there are two subunits each of HSD17B8 (for example, chains A and D) and CBR4 (chains B and C) ( Fig. 2b ). Therefore, the Hs KAR heterotetramer is essentially a dimer of HSD17B8 and CBR4 dimers ( Fig. 2b ) with approximate 222 (D2) symmetry, resembling the previously studied homotetrameric KARs. Although the overall structures of the two molecules of HSD17B8 and CBR4 in a tetramer are very similar, there are subtle differences between these chains such that each chain can be uniquely identified in each of the four tetramers of the asymmetric unit. Two subunits of HSD17B8 (or CBR4) interact with each other through helices α4 and α5, forming a four-helix bundle ( Fig. 2b ). At the interaction surface between HSD17B8 and CBR4, the corresponding β7 β-strands from each subunit associate in an anti-parallel manner interacting through water-mediated H-bonds, forming an extended continuous β-sheet ( Fig. 2b ). Two helices (α6) from both subunits are also packed against each other. The structure of homotetrameric Hs HSD17B8 (PDB id: 2PD6) is known. However, when Hs HSD17B8 and Hs CBR4 are co-expressed, they always form heterotetramers. Analysis of the interfaces by the web-based PDBePISA [21] (Protein interfaces, surfaces and assemblies’ service at the European Bioinformatics Institute: http://www.ebi.ac.uk/pdbe/prot_int/pistart.html ) shows that the homodimeric interfaces (for example, the AD and BC interfaces) in Hs HSD17B8 and Hs KAR-NAD(P) + structures are comparable (~1,600 Å 2 ). However, each heterodimeric interface in Hs KAR (for example, the AB and DC interface) is ~200 Å 2 larger than the corresponding interface in the homotetrameric Hs HSD17B8 ( Fig. 2b and Supplementary Table 1 ). Moreover, the diagonally opposite protomers in the Hs KAR tetramer (AC and DB interface) also have an interface of ~200 Å 2 each, whereas there is no interaction between the corresponding protomers in the Hs HSD17B8 homotetramer ( Supplementary Fig. 2 ). Together, these additional interfaces amount to ~800 Å 2 , leading to a stabilization of the heterotetramer by ~8 kcal mol −1 according to the PISA calculations. In addition, a hypothetical homotetramer of Hs CBR4 shows many steric clashes between the carboxy terminus of the two diagonally opposite protomers (that is, AC and DB interface). Therefore, the heteotetrameric assembly of Hs HSD17B8 and Hs CBR4 as seen in our crystal structure of Hs KAR is much more favourable than the corresponding homotetramers. Cofactor recognition and the catalytic triad in Hs KAR The crystals of Hs KAR could only be obtained when cocrystallized with 2 mM NAD + . In the crystal structure, NAD + is bound only to the HSD17B8 subunits and the CBR4 subunits are in the apo form. Several attempts to crystallize Hs KAR in the apo form as well as in the presence of other ligands such as coenzyme A (CoA), NADP + , NADH and NADPH were not successful. Therefore, we soaked the crystals of Hs KAR-NAD + with a mixture of 5 mM each of NAD + and NADP + in the crystallization solution. The resulting structure showed the selective binding of NAD + to the HSD17B8 subunits and of NADP + to the CBR4 subunits. The 2′-phosphate moiety was unambiguously visible in the initial omit maps ( Fig. 2c ), demonstrating the cofactor preference of the two subunits. The conformation of NAD + and NADP + in the respective binding sites are similar to that of NADP + in Brassica napus ( B. napus) and E. coli fabG [13] , [15] . Both NAD + and NADP + are stabilized by many conserved hydrogen bonding interactions in their respective binding sites ( Fig. 2c and Supplementary Table 2 ). The differences are mainly due to the presence of the 2′-phosphate moiety of NADP + . In HSD17B8, the side chain of αAsp42 (residues of HSD17B8 and CBR4 subunits are represented with the prefix α and β, respectively) has two key hydrogen bonding interactions with the two oxygen atoms (O2B, 2.5 Å and O3B, 2.7 Å) of the ribose moiety of the adenosine part of NAD + ( Fig. 2c and Supplementary Table 2 ). This is a conserved interaction in many NAD + binding enzymes [22] . The αAsp42 is replaced by βAla33 in the NADP(H)-specific Hs CBR4 providing enough space for the additional 2′-phosphate moiety of NADP + . This phosphate group is stabilized in its position by hydrogen bonding interactions from βArg12 (3.5 Å) and βArg34 (2.7 Å) ( Fig. 2c ). Therefore, αAsp42, βArg12 and βArg34 are crucial for the cofactor recognition and differentiation. In an Hs KAR tetramer, NAD + is bound equally well in both the HSD17B8 subunits, whereas the nicotinamide part of NADP + is disordered in one of the two CBR4 subunits (chain C, for example). Structural and sequence comparisons suggest that in Hs HSD17B8 αSer156, αTyr169 and αLys173, and in Hs CBR4 βSer135, βTyr148 and βLys152 are the catalytic triad residues involved in catalysis ( Fig. 3a ) [13] , [23] . The side chains of these residues can be clearly identified and are positioned near the nicotinamide moiety ( Fig. 2c ). αTyr169 and αLys173 of HSD17B8 and the corresponding residues (βTyr148 and βLys152) of CBR4 have hydrogen bonding interactions with the ribose oxygen (O2D, 3.2 Å and 2.7 Å) of the nictotinamide part of NAD(P) + . The catalytic serine (αSer156 and βSer135) is proposed to provide an oxyanion hole for the thioester oxygen of the substrate [24] . Interestingly, this serine in many of the subunits shows electron density extended beyond its side chain. The shape of this density is varied. For example, in chain D, the αSer156 is modelled as O -acetylserine (Oas), whereas in chain M an acetate ion and a water molecule can be modelled unambiguously ( Supplementary Fig. 3 ). In chains H and P, the density is ambiguous although an acetate ion is modelled there. All these chains represent HSD17B8 subunits. In other chains, a water molecule is sufficient to account for the observed extra density. Only in chain O (CBR4 subunit), there is still some spurious positive density, which could not be modelled. The cause of the different behaviour of this serine in different subunits of Hs KAR is unclear. Subtle crystal packing effects could be one of the reasons. The modelled acetate ion is near the nicotinamide ring of NAD + and to some extent identifies the fatty-acyl chain binding pocket. The sodium acetate buffer and the ammonium acetate used in the crystallization condition can be the source of these acetate ions. Acetylated serine is also observed in a few other crystal structures, which are either acetyltransferases or esterases where ligands such as acetyl-CoA or acetylcholine are used [25] , [26] . There is one protein structure of acetylxylan esterase (PDB id: 3FYU, Krastanova et al. , unpublished) crystalized in the presence of 0.2 M sodium acetate and xylan containing acetylated catalytic [27] serines. Similar to that in Hs KAR, the serine is acetylated only in some subunits. 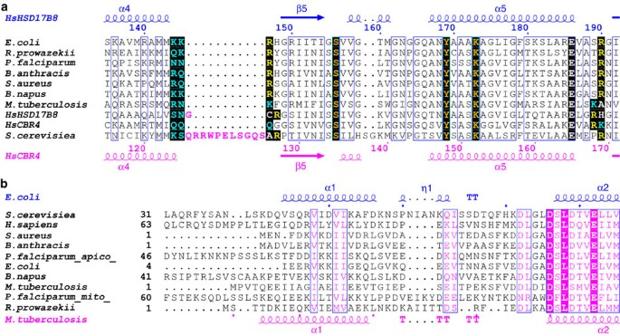Figure 3: Sequence alignment of KARs and ACPs. (a) Part of the sequence alignment ofHsHSD17B8 andHsCBR4 ofHsKAR with KAR orthologues. The secondary structure elements as calculated by DSSP and residue numbers are displayed above forHsHSD17B8 and below forHsCBR4. The conserved catalytic triad residues, Ser-Tyr-Lys are highlighted in orange. The arginine residues close to Arg129 and Arg172 inE. colifabG essential for ACP binding are highlighted in yellow. The extended loop inS. cerevisiae Oar1 near Arg129 ofE. colifabG is shown in magenta. Other positively charged residues near this region are highlighted in cyan. The full sequence alignment can be found in theSupplementary Fig. 1. (b) Part of the sequence alignment of ACPs from the same organisms as inFig. 3a. The secondary structure elements above and below the sequences correspond to ACP fromE. coliandM. tuberculosis, respectively. It can be seen that the helix α2, considered to be essential for the interaction with KAR, is quite well conserved in these organisms, in particular with respect to the two negatively charged residues (Asp76 and Glu82,E. coliACP numbering). The full sequence alignment is provided in theSupplementary Fig. 5. Figure 3: Sequence alignment of KARs and ACPs. ( a ) Part of the sequence alignment of Hs HSD17B8 and Hs CBR4 of Hs KAR with KAR orthologues. The secondary structure elements as calculated by DSSP and residue numbers are displayed above for Hs HSD17B8 and below for Hs CBR4. The conserved catalytic triad residues, Ser-Tyr-Lys are highlighted in orange. The arginine residues close to Arg129 and Arg172 in E. coli fabG essential for ACP binding are highlighted in yellow. The extended loop in S. cerevisi ae Oar1 near Arg129 of E. coli fabG is shown in magenta. Other positively charged residues near this region are highlighted in cyan. The full sequence alignment can be found in the Supplementary Fig. 1 . ( b ) Part of the sequence alignment of ACPs from the same organisms as in Fig. 3a . The secondary structure elements above and below the sequences correspond to ACP from E. coli and M. tuberculosis , respectively. It can be seen that the helix α2, considered to be essential for the interaction with KAR, is quite well conserved in these organisms, in particular with respect to the two negatively charged residues (Asp76 and Glu82, E. coli ACP numbering). The full sequence alignment is provided in the Supplementary Fig. 5 . Full size image Enzymological studies of Hs KAR and its active site variants A number of residues near the catalytic sites were targeted for mutagenesis in both HSD17B8 and CBR4 ( Fig. 2c , and Supplementary Tables 3 and 4 ). Large-scale purification was attempted for all of these mutants. However, only purified samples of αD42A- Hs KAR, αY169A- Hs KAR, αK173A- Hs KAR, βR34A- Hs KAR and βK152A- Hs KAR could be prepared following a protocol similar to that of the Hs KAR purification. The reductase enzyme activities of Hs KAR and mutated derivatives thereof were tested in vitro with acetoacetyl-CoA and 9,10-phenanthrene quinone (9,10-PQ) in the presence of NAD(P)H. The calculated specific activities and relative activities of these variants with respect to Hs KAR are listed in Table 2 . Overall, the specific activity was higher for Hs KAR in the presence of NADH (21 μmol mg −1 min −1 for both the substrates) in comparison with the NADPH-dependent activity of 0.7 and 2.6 μmol mg −1 min −1 for acetoacetyl-CoA and 9,10-PQ, respectively. A substantial loss of NADH-dependent activity was observed for the HSD17B8 active site mutants. The αY169A- Hs KAR shows specific activity of 0.65 and 0.85 μmol mg −1 min −1 with acetoacetyl-CoA and 9,10-PQ, respectively. Similarly, the respective specific activities for the αK173A- Hs KAR are 0.06 and 1.2 μmol mg −1 min −1 . In contrast, the βK152A- Hs KAR and βR34A- Hs KAR mutants of CBR4 subunit did not lose any NADH-dependent activity. The activity profile was opposite when NADPH was used as the cofactor. In particular, this trend was clearly visible with the substrate 9,10-PQ. With NADPH, the HSD17B8 active site mutants (αY169A and αK173A- Hs KAR) are as active as the wild-type Hs KAR, whereas the CBR4 mutants (βR34A and βK152A- Hs KAR) showed reduced activity ( Table 2 ). The βR34A- Hs KAR mutant kept only about 13% and 17% of the NADPH-dependent Hs KAR activity with acetoacetyl-CoA and 9,10-PQ, respectively. The βK152A- Hs KAR did not display any measurable NADPH-dependent activity with acetoacetyl CoA but with 9,10-PQ, this mutant had 18% of the corresponding Hs KAR activity. Table 2 Specific activity of Hs KAR and its mutated variants. Full size table The αD42A- Hs KAR variant shows reduced activity of ~36% and 22% with NADH when compared with the wild-type Hs KAR using acetoacetyl-CoA and 9,10-PQ as the substrates, respectively. However, there was a significant increase (~500%) of NADPH-dependent activity in comparison with the native enzyme. When αAsp42 is mutated to a smaller residue such as alanine, it apparently provides sufficient space for the 2′-phosphate group of NADPH to bind. As a result, the mutated HSD17B8 subunit cofactor binding site might be able to accommodate NADPH to some extent, leading to higher NADPH-dependent activity of αD42A- Hs KAR. These data reinforce the conclusion that the NADH-dependent activity can be mapped to the HSD17B8 active site and the NADPH-dependent activity to the CBR4 subunit in Hs KAR. In addition, these data show that HSD17B8 has higher catalytic activity compared with CBR4 ( Table 2 ), at least under the tested conditions with the available substrates. Moreover, it can be noted that HSD17B8 has much higher quinone reductase activity than CBR4, which has been described as a quinone reductase. It is probable that the observed quinone reductase activity of CBR4 is not physiologically significant and the primary role of CBR4 may not be related to its quinone reductase activity. SPR binding studies To better understand the phenomenon of cofactor recognition by Hs KAR, we determined the binding affinities for the cofactors by SPR. The kinetics of the cofactor binding could not be studied as the association and dissociation of the cofactors were too fast and gave only square pulses ( Supplementary Fig. 4 ). These measurements show that NADPH has the highest binding affinity followed by NADP + , NADH and NAD + ( Supplementary Table 5 ). 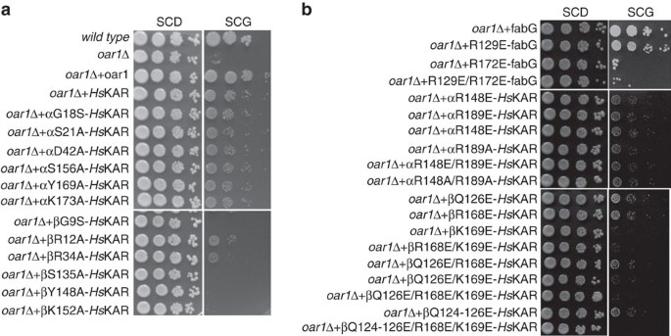Figure 5: Spotting assays for wild-type andOAR1-deficient yeast in SC media with glucose (D) or glycerol (G) as the sole carbon source. (a) Transformation with plasmids harbouringOAR1orHsKAR genes can rescue the growth of yeast in glycerol medium. These assays show that the mutations in the active site ofHsHSD17B8 (α) subunit do not affect the complementation ofHsKAR (top panels), whereas the mutations in theHsCBR4 (β) subunit destroy the yeast complementation properties ofHsKAR (bottom panels). This reveals the importance of the NADPH-dependent CBR4 subunit in ‘in vivo’KAR activity. (b) Similar spotting assays for variants ofE. coli fabG(top panels), HSD17B8 variants (middle panels) and CBR4 variants (bottom panels) of the residues proposed to be involved in ACP recognition. These assays reveal the physiological significance of Arg172 of theE. colifabG in the recognition of ACP (top panels). Growth of HSD17B8 variants are not affected, indicating they are not involved in ACP recognition (middle panels). The key residue for the ACP recognition is βLys169 of CBR4, as all the variants containing this mutation cannot complement theoar1deletion in yeast (bottom panels). These experiments also show that NADH and NADPH have two binding sites with differing affinities ( Fig. 4 ). In the stronger binding site of NADPH, the affinity is in the micromolar range ( K D =8.2 μM), whereas the weaker (second) binding site affinity is in the millimolar range (8.6 mM). Similarly, the strong and weak binding site affinities for NADH are 33.4 μM and 20.4 mM, respectively. For both these cofactors, ligand concentrations up to 40 mM were used in the SPR measurements. However, for NADP + and NAD + , measurements beyond 5 mM were not of good quality. Therefore, although NADP + showed some signs of dual site binding, only the stronger binding affinity with a K D value of 26.8 μM could be determined. NAD + has a K D value of 4.2 mM, the lowest affinity among the tested ligands. 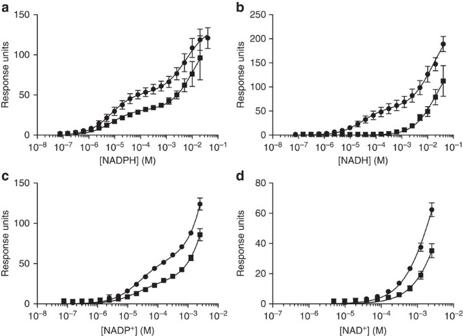There is no evidence for a second binding site. Figure 4: Binding studies withHsKAR and αD42A-HsKAR. Relative SPR responses for the binding of (a) NADPH, (b) NADH, (c) NADP+and (d) NAD+toHsKAR are shown in dots (•) and to αD42A-HsKAR are shown in squares (▪). Each experiment was repeated at least three times and the error bars indicate the s.d. The concentration on thexaxis is plotted on a logarithmic scale to visualize the two site binding observed for NADPH and NADH. It is evident that the high-affinity binding site is not present for NADH with αD42A-HsKAR. The curves fitted by nonlinear regression using two-site or one-site specific binding module of the Graphpad Prism software are shown in black. The figure was prepared using the Graphpad Prism software. The binding affinities are listed inSupplementary Table 5. Figure 4: Binding studies with Hs KAR and αD42A- Hs KAR. Relative SPR responses for the binding of ( a ) NADPH, ( b ) NADH, ( c ) NADP + and ( d ) NAD + to Hs KAR are shown in dots (•) and to αD42A- Hs KAR are shown in squares (▪). Each experiment was repeated at least three times and the error bars indicate the s.d. The concentration on the x axis is plotted on a logarithmic scale to visualize the two site binding observed for NADPH and NADH. It is evident that the high-affinity binding site is not present for NADH with αD42A- Hs KAR. The curves fitted by nonlinear regression using two-site or one-site specific binding module of the Graphpad Prism software are shown in black. The figure was prepared using the Graphpad Prism software. The binding affinities are listed in Supplementary Table 5 . Full size image Our crystallographic and enzymological studies clearly demonstrate the cofactor specificity of HSD17B8 and CBR4 to be NAD(H) and NADP(H), respectively. Therefore, there are two NAD(H) and two NADP(H) binding sites in Hs KAR. Assuming that all of the immobilized protein is active, the theoretically calculated binding level in response units (RUs) for the binding of one ligand molecule to the Hs KAR tetramer is ~60 RU. This is in agreement with the experimentally observed RU for the stronger binding affinity (53±5 RU for NADPH and 53±9 RU for NADH). Therefore, the number of binding sites for either NADH or NADPH with micromolar affinity is one per Hs KAR tetramer. It is possible that NADH (or NADPH) binds to one of the two molecules of HSD17B8 (or CBR4) with micromolar affinity and that this binding reduces the affinity of the second binding site to millimolar levels, which would be a case of negative cooperativity. However, in our crystal structure we do not observe significant structural variation between the two binding sites. The main difference is that the nicotinamide part of NADP + is disordered in one of the CBR4 subunits of each tetramer. Negative cooperativity of cofactor binding has been observed in E. coli [14] and Plasmodium falciparum ( P. falciparum ) [28] fabGs in particular in the presence of ACP. Therefore, the mechanism of cooperativity in Hs KAR could differ from that observed in E. coli [14] and P. falciparum FabG [28] . At this point, we do not know how ACP affects the cofactor binding for Hs KAR. Moreover, positive cooperativity has been observed for Mycobacterium tuberculosis ( M. tuberculosis ) [29] and Staphylococcus aureus fabGs [20] even in the absence of ACP. We also determined the binding affinities for the αD42A- Hs KAR mutant. For this variant, the NAD + binding affinity decreased by ~15-fold with a K D value of 70.8 mM. The high-affinity binding site of NADH was also abolished in this mutant exhibiting single-site binding with a K D value of 15 mM. However, the association with NADPH or NADP + was not affected ( Supplementary Table 5 ), demonstrating the importance of αAsp42 to differentiate between NAD(H) and NADP(H) binding [14] , [20] . In vivo functional analysis To evaluate the physiological significance of the two subunits of Hs KAR, we set up a yeast complementation assay taking advantage of the dependence of yeast cells on a functional mitochondrial KAR for respiratory competence. Wild-type yeast cells can grow very well on either glucose or glycerol as the sole carbon source, while cells deficient of the OAR1 , the gene encoding the native yeast mitochondrial KAR, survive only on fermentable media. To rescue the growth of oar1Δ cells on glycerol-based plates, the OAR1 (or fabG or HsKAR ) gene has to be transformed into the cells to complement the deficiency. Therefore, it is possible to use yeast as an in vivo system to evaluate the effects of the Hs KAR mutant variants on respiratory growth. Intriguingly, these studies show that mutations at the NAD(H) binding and catalytic sites of the HSD17B8 of Hs KAR did not affect the growth of the cells on synthetic complete (SC)-glycerol plates. However, NADP(H)-binding site and catalytic site mutant variants of CBR4 (residues βGly9, βSer135, βTyr148 and βLys152; Supplementary Table 4 ) are unable to support respiratory growth ( Fig. 5a ). This shows that CBR4 is the catalytic subunit carrying the KAR activity that is physiologically relevant in vivo for the complementation of the yeast mtFAS defect. Figure 5: Spotting assays for wild-type and OAR1 -deficient yeast in SC media with glucose (D) or glycerol (G) as the sole carbon source. ( a ) Transformation with plasmids harbouring OAR1 or Hs KAR genes can rescue the growth of yeast in glycerol medium. These assays show that the mutations in the active site of Hs HSD17B8 (α) subunit do not affect the complementation of Hs KAR (top panels), whereas the mutations in the Hs CBR4 (β) subunit destroy the yeast complementation properties of Hs KAR (bottom panels). This reveals the importance of the NADPH-dependent CBR4 subunit in ‘ in vivo’ KAR activity. ( b ) Similar spotting assays for variants of E. coli fabG (top panels), HSD17B8 variants (middle panels) and CBR4 variants (bottom panels) of the residues proposed to be involved in ACP recognition. These assays reveal the physiological significance of Arg172 of the E. coli fabG in the recognition of ACP (top panels). Growth of HSD17B8 variants are not affected, indicating they are not involved in ACP recognition (middle panels). The key residue for the ACP recognition is βLys169 of CBR4, as all the variants containing this mutation cannot complement the oar1 deletion in yeast (bottom panels). Full size image In vivo ACP recognition by Hs KAR For mtFAS, the substrates are fatty acyl conjugates of ACP, similar to that for bacterial FAS-II. ACP is highly conserved in amino acid sequence, especially, the helix α2, which is at the ACP-enzyme interaction site [30] . The identity of amino acid sequences of the helix α2 between E. coli , Saccharomyces cerevisiae ( S. cerevisiae ) and human is 70% ( Fig. 3b and Supplementary Fig. 5 ). In E. coli fabG, two arginine residues, Arg129 and Arg172, were found to play an important role in ACP recognition and binding [30] . In enzyme activity assays, E. coli fabG variants fabG-R129E and fabG-R172E showed 8.5% and 3.5% of ACP-dependent activity, respectively, while CoA-dependent activities were largely unaffected [30] . These arginines are well conserved in most of the fabG-type enzymes. However, in M. tuberculosis , yeast and Hs KAR, they are not strictly maintained. In Hs HSD17B8, there are two arginine residues Arg148 and Arg189 that are not exactly in the same positions as Arg129 and Arg172 of E. coli fabG, but in the neighbouring sites ( Fig. 3a ). In CBR4, βGln126 and βLys169 are located in the position corresponding to Arg129 and Arg172 of E. coli fabG, respectively. In CBR4, there is also an arginine (βArg168) in a position adjacent to that of Arg172 of E. coli fabG ( Fig. 3a ). These residue changes could affect ACP binding in subtle ways. In both HSD17B8 and CBR4, these residues are on the surface pointing into bulk solvent and are far away from the catalytic site of the same subunit. A superposition of the Hs KAR structure and the ternary complex of M. tuberculosis fabG4 with bound NAD + and hexanoyl-CoA [31] showed the probable fatty-acyl binding pocket in both HSD17B8 and CBR4. 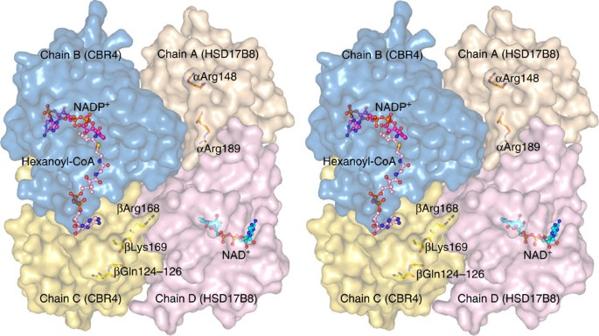Figure 6: Stereo diagram of theHsKAR tetramer in surface representation highlighting the residues chosen for mutation to study the ACP recognition. The chosen residues are represented as sticks on chain C (yellow; CBR4) and chain A (brown; HSD17B8). NADP+is shown bound in chain B (magenta ball-and-stick). The pink ball-and-stick model is hexanoyl-CoA fromM. tuberculosisfabG4 (PDB id: 3V1U) superposed onHsKAR (CBR4; chain B) to show the predicted fatty-acyl and pantetheine binding groove ofHsKAR extending from CBR4 chain B to CBR4 chain C. Thein vivodata indicate that the ACP conjugated to the fatty acyl tail binds to the CBR4 subunit (chain C) near βLys169. Figure 6 illustrates the relative positions of the proposed ACP-recognition residues of HSD17B8 (chain A) and CBR4 (chain C) with respect to the neighbouring active site of CBR4 (chain B). This arrangement suggests two possibilities for ACP binding: the ACP interacts with Hs KAR either (i) through the residues on the surface of CBR4 (chain C) and extend the fatty acyl chain to the active site of neighbouring CBR4 subunit (chain B) in a similar manner as in Fig. 6 or (ii) through the surface residues of HSD17B8 (chain A) and extend the fatty acyl chain through another groove to the CBR4 active site (chain B). To experimentally test these predictions, we created a number of single and multiple mutated variants of Hs KAR ( Supplementary Tables 3 and 4 ). Figure 6: Stereo diagram of the Hs KAR tetramer in surface representation highlighting the residues chosen for mutation to study the ACP recognition. The chosen residues are represented as sticks on chain C (yellow; CBR4) and chain A (brown; HSD17B8). NADP + is shown bound in chain B (magenta ball-and-stick). The pink ball-and-stick model is hexanoyl-CoA from M. tuberculosis fabG4 (PDB id: 3V1U) superposed on Hs KAR (CBR4; chain B) to show the predicted fatty-acyl and pantetheine binding groove of Hs KAR extending from CBR4 chain B to CBR4 chain C. The in vivo data indicate that the ACP conjugated to the fatty acyl tail binds to the CBR4 subunit (chain C) near βLys169. Full size image The arginine residues Arg129 and Arg172 in E. coli fabG have been demonstrated to be involved in ACP binding only by in vitro tests [30] . Therefore, the variants fabG-R129E and fabG-R172E of E. coli fabG were re-investigated using our yeast in vivo system ( Fig. 5b ). These experiments confirmed that Arg172 is very likely to play a critical role in the fabG-ACP recognition in vivo as the fabG-R172E variant showed very poor growth on SC glycerol media. In contrast, the fabG-R129E variant did not severely affect the growth of the yeast cells. The corresponding Hs KAR single and multiple mutant variants were also evaluated using the same system. The mutations of the HSD17B8 subunit did not impact on the growth of the yeast cells ( Fig. 5b ). However, the CBR4 βK169E mutation affected growth, suggesting that βLys169 of CBR4 in Hs KAR is critical for ACP recognition. Single, double and triple mutants carrying this variant (βK169E-, βQ126E/βK169E- and βQ126E/R168E/K169E- Hs KAR, respectively) and additional single mutant (βR168E- Hs KAR) were expressed in E. coli , purified and their specific activities measured ( Table 2 ). The single and double mutants show CoA-dependent specific activities comparable to the wild-type Hs KAR. Only the triple mutant shows reduced (14% remaining) NADPH-dependent activity. These results suggest that the mutation of βLys169 to Glu does not affect the folding, stability and CoA-dependent activity of Hs KAR, but disrupts the ability to recognize ACP in vivo . It can be noted here that βLys169 of Hs KAR is in the same position as Arg172 of E. coli fabG ( Fig. 3a ). Therefore, our yeast complementation studies clearly demonstrate that CBR4 is the catalytic as well as the ACP-binding subunit of Hs KAR for the mtFAS activity. The importance of the mtFAS pathway has recently been recognized, as it is related to lipoic acid synthesis [32] , [33] , diseases such as cardiomyopathy in mammals [34] , mitochondrial respirational dysfunction and accelerated aging [33] . Hs KAR, one of the enzymes of this essential mtFAS pathway, is a unique heterotetramer formed by Hs HSD17B8 and Hs CBR4 (ref. 9 ). In this study, we show that the reductase activity of the Hs CBR4 (β-subunit) is NADPH-dependent and responsible for the KAR activity of mtFAS. These data, for the first time, give a clue on the physiological function of CBR4. Hs HSD17B8, the α-subunit of Hs KAR, is NAD(H)-dependent and is necessary for a soluble and competent complex. As discussed further below, we speculate on a possible role for this subunit in routing the 3R-hydroxyacyl-CoA intermediates emerging from the metabolism of unsaturated fatty acids to the mitochondrial β-oxidation pathway. The Hs KAR crystal structures show that Hs HSD17B8 and H sCBR4 form a physically interacting and functional Hs KAR α 2 β 2 -tetramer. These results are in agreement with our previous study demonstrating that co-expression of Hs HSD17B8 and Hs CBR4 in the oar1Δ yeast cells rescues their growth on a non-fermentable carbon source. Purification experiments demonstrate that HSD17B8 only forms heterotetramers with CBR4 on heterologous co-expression in E. coli [9] . Our attempts to purify the homotetrameric Hs HSD17B8 and Hs CBR4 separately resulted in very low protein yield due to their poor solubility compared with the heterotetrameric Hs KAR. Nevertheless, the deposited structure of Hs HSD17B8 (PDB id: 2PD6) shows that this protein can form homotetramers in the absence of CBR4. The observed heterotetrameric arrangement of Hs KAR is similar to the homotetrameric orthologues of Hs KAR, for example, from B. napus and E. coli [13] , [14] , and the two subunits interact in an optimal way, providing higher stability to the heterotetramer than to the respective homotetramers. The enzyme kinetic data define the distinctive functionalities of the HSD17B8 and CBR4 subunits of Hs KAR. Mutations in the HSD17B8 active site (αY169A and αK173A- Hs KAR) specifically reduce much the NADH-dependent activities, while mutations in the CBR4 catalytic site (βK152A- Hs KAR) affect only the NADPH-dependent activities ( Table 2 ). The SPR binding studies show that NADPH has the highest affinity for Hs KAR. In addition, NADPH and NADH showed a weak-affinity second binding site with K D in the millimolar range, which may be due to negative cooperativity in Hs KAR. SPR binding studies with the αD42A- Hs KAR variant show that the NAD(H) binding is affected. These data, together with our crystallographic binding studies, show the selective recognition of NAD(H) and NADP(H) by the Hs HSD17B8 and Hs CBR4 subunits of the Hs KAR complex, respectively. The in vivo role of the NADPH-dependent CBR4 subunit of Hs KAR is immediately evident from our yeast complementation experiments with Hs KAR. These studies clearly show that mutations at the CBR4 active site impair the growth in the presence of glycerol, while the growth of the HSD17B8 mutants is the same as for the wild-type cells. This implies that CBR4 is the catalytically active subunit with respect to the mtFAS KAR activity, and the cofactor for the mtFAS is NADPH ( Fig. 1 ) as also observed in other FAS-II pathways. As the reactions of mtFAS use thioesters of ACP as substrates, we assessed the role of Hs KAR subunits in ACP recognition through mutagenesis and yeast complementation studies. These studies show that only the CBR4 variants of Hs KAR containing the mutation βK169E were unable to rescue the growth of the oar1Δ yeast cells on glycerol as the sole carbon source, suggesting that βLys169 is involved in ACP recognition. These experiments provide credence that CBR4 is responsible for both the catalytic activity associated with mtFAS pathway as well as ACP-recognition ( Fig. 7 ). The relatively low catalytic activity of the NADPH-dependent CBR4 might also be due to the fact that the real substrate is the fatty-acyl-ACP conjugate. 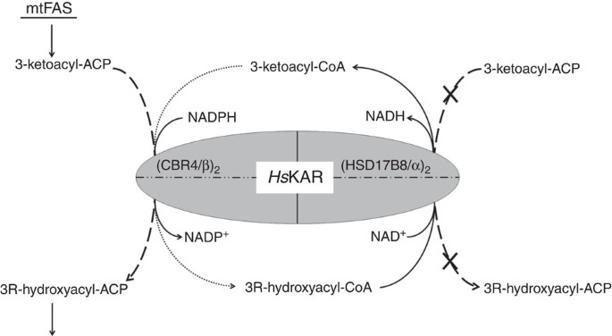Figure 7: Schematic representation of the catalytic properties of theHsKAR subunits (CBR4 (β) and HSD17B8 (α)) in the context of the mtFAS pathwayin vivo. The CBR4 subunit is the functional subunit of the KAR complex catalysing the conversion of 3-ketoacyl-ACP to 3R-hydroxyacyl-ACP (dashed arrow). CBR4 is a poor acceptor of fatty acyl-CoA conjugates (dotted arrow). The high affinity of the CBR4 subunit for NADPH will favour the reduction of 3-ketoacyl-ACP to 3R-hydroxyacyl-ACP whenever the NADPH/NADP+ratio is high. The HSD17B8 subunit may not accept fatty acyl-ACP conjugates (dashed arrow with cross). However, the HSD17B8 subunit does efficiently catalyse the NAD+-dependent conversion of 3R-hydroxyacyl-CoA into 3-ketoacyl-CoA, and therefore can introduce 3R-hydroxyacyl-CoA into the mitochondrial β-oxidation pool. Figure 7: Schematic representation of the catalytic properties of the Hs KAR subunits (CBR4 (β) and HSD17B8 (α)) in the context of the mtFAS pathway in vivo . The CBR4 subunit is the functional subunit of the KAR complex catalysing the conversion of 3-ketoacyl-ACP to 3R-hydroxyacyl-ACP (dashed arrow). CBR4 is a poor acceptor of fatty acyl-CoA conjugates (dotted arrow). The high affinity of the CBR4 subunit for NADPH will favour the reduction of 3-ketoacyl-ACP to 3R-hydroxyacyl-ACP whenever the NADPH/NADP + ratio is high. The HSD17B8 subunit may not accept fatty acyl-ACP conjugates (dashed arrow with cross). However, the HSD17B8 subunit does efficiently catalyse the NAD + -dependent conversion of 3R-hydroxyacyl-CoA into 3-ketoacyl-CoA, and therefore can introduce 3R-hydroxyacyl-CoA into the mitochondrial β-oxidation pool. Full size image The current data show that the CBR4 subunit of Hs KAR is essential for complementation of the oar1 Δ respiratory deficient phenotype in vivo in yeast. In the cytosolic FAS-I complex, KAR is composed of a catalytic and a non-catalytic domain (ψKAR), the latter providing only a structural role [35] . HSD17B8 may serve an analogous purpose. This is also supported by the observations that the Hs KAR α 2 β 2 -tetramer possesses much higher solubility than when CBR4 is expressed alone, and that a hypothetical CBR4 tetramer shows many steric clashes mainly between the C terminus of diagonally opposite protomers in the tetramer. However, apart from being essential for the formation of a competent α 2 β 2 -complex, it is intriguing to note that the HSD17B8 subunit is highly active in the reductive (this study) as well as dehydrogenating direction as shown by us in a previous study [9] unlike the non-catalytic ψKAR domain of the FAS-I complex. This indicates that the function of the HSD17B8 subunit in Hs KAR is not limited to just a structural role. The mitochondrial NADPH and NAD + concentrations are in the millimolar range [36] , [37] and are much higher than the concentration of NADP + and NADH [38] under conditions pertaining in the coupled respiring mammalian mitochondria favouring the NADPH-dependent fatty acid synthesis and the NAD + -dependent β-oxidation. Therefore, in mitochondria, the NADP(H)-dependent CBR4 subunit of Hs KAR works in reductive direction for fatty acid synthesis and the NAD(H)-dependent HSD17B8 subunit can work towards the dehydrogenating direction. Curiously, the NAD + -dependent dehydrogenase reaction of HSD17B8 is specific for 3R-hydroxyacyl-CoA [9] . In peroxisomes, the 3R-hydroxyacyl-CoA intermediates are metabolized by a homologue of HSD17B8, the NAD + -dependent hydratase domain of the multifunctional enzyme, type-2 (ref. 39 ). In mitochondria, β-oxidation proceeds via 3S-hydroxyacyl-CoA intermediates. A probable source of 3R-hydroxyacyl-CoA intermediates in mitochondria is the β-oxidation of polyunsaturated fatty acids (PUFAs). The unsaturated intermediates of Z-PUFAs are converted to 2E-enoyl-CoA with the help of the auxiliary enzymes of mitochondrial β-oxidation, Δ 3,5 , Δ 2,4 -dienoyl-CoA isomerase, Δ 3,2 -enoyl-CoA isomerase and Δ 2,4 -dienoyl-CoA reductase [40] . However, if Z-PUFAs escape this auxiliary pathway, then 2Z-enoyl-CoA metabolites are formed. In mitochondria, these are converted to 3R-hydroxyacyl-CoA esters by enoyl-CoA hydratase 1 (ref. 41 ). Under such conditions, HSD17B8 of the Hs KAR complex can prevent the accumulation of these intermediates by efficient conversion of 3R-hydroxyacyl-CoA to 3-ketoacyl-CoA. Therefore, we speculate that this HSD17B8 catalytic activity may act as a rescue route reintroducing 3R-hydroxyacyl-CoA esters into the mitochondrial β-oxidation intermediate pool ( Fig. 7 ), functioning as a fourth auxiliary enzyme of the mitochondrial β-oxidation pathway. We have initiated studies to test this function in vivo in suitable genetically modified mouse models. Media and strains Yeast ( S. cerevisiae ) cells were grown either on YPD (1% yeast extract, 2% peptone and 2% D-glucose), YPG (1% yeast extract, 2% peptone and 3% glycerol) or SC medium (Sigma-Aldrich, Helsinki, Finland), SC-glucose (2%), SC-glycerol (3%), or other SC medium lacking one or more nutrients. The yeast and bacterial strains used in this study are listed in Supplementary Table 6 . The BY4741 oar1 Δ strain was obtained from EUROSCARF (Frankfurt, Germany). Molecular cloning and site-directed mutagenesis The oligonucleotides used are listed in Supplementary Table 3 . PCR amplification were carried out using Pfu polymerase (Stratagene, La Jolla, CA, USA). The p631- Hs KAR construct for the bacterial protein production and YEp- Hs KAR construct for yeast complementation experiments expressing Hs KAR components Hs HSD17B8 and Hs CBR4 (ref. 9 ) were used as templates for generating mutated variants by applying a QuickChange site-directed mutagenizes kit (Stratagene). Mutations were verified by sequencing and the plasmids encoding mutants were transformed into BL21 (RARE) E. coli cells for protein synthesis or yeast BY4741 oar1 Δ cells for complementation assays. Protein expression and purification p631- Hs KAR and its mutant variants were expressed and purified by following a similar protocol [9] . Briefly, BL21 (RARE) cells containing plasmids were cultured in M9ZB medium at 37 °C until OD 600 reach 0.6. 0.1 mM isopropyl-β- D -thiogalactoside was then added into the media and cells were incubated at 18 °C for additional 18–20 h. The collected cells were resuspended in 20 mM Tris buffer with 500 mM sodium chloride, 5 mM imidazole, 10% glycerol and 0.1% Triton-X 100 at pH 7.9, sonicated, and Hs KAR was purified by Ni-NTA affinity chromatography from the soluble fraction using a buffer containing 20 mM Tris, 500 mM sodium chloride pH 7.9 and 5–500 mM imidazole. The fractions containing Hs KAR were then pooled and loaded for further purification onto a Superdex 200 size-exclusion chromatography column (GE Healthcare, New York, USA) previously equilibrated with 20 mM HEPES buffer pH 7.2 containing 120 mM potassium chloride, 1 mM EDTA and 1 mM sodium azide. The purified protein was concentrated and stored at −70 °C until used further. Crystallization and structure determination Hs KAR was crystallized using the sitting drop vapour diffusion method at room temperature. One microlitre of Hs KAR at a concentration of 8 mg ml −1 with 2 mM NAD + was mixed with 1 μl of the crystallization solution containing 15–18% PEG3350 and 0.4 M ammonium acetate in sodium acetate buffer at pH 5.0. Hs KAR crystals appeared in 1–2 weeks. The crystals of Hs KAR complexed with both NAD + and NADP + were obtained by soaking the crystals co-crystallized with NAD + in a solution containing the crystallization condition with additional 5 mM NAD + and 5 mM NADP + overnight. Before data collection, the crystals were transferred into a crystallization solution containing also 20% ethylene glycol as the cryo-protectant and subsequently were frozen in liquid nitrogen. X-ray diffraction data of the Hs KAR-NAD + complex crystals were collected at the European Synchrotron Radiation Facility, Grenoble, France, beamline ID-29 at a wavelength of 0.9763 Å using the ADSC Quantum Q315r detector. The data were processed with the iMOSFLM [42] and XDS [43] packages. Twinning was detected and the twin fraction was calculated by Phenix.xtriage [44] . There are four tetramers per asymmetric unit. The data collection statistics are given in Table 1 . The structure was solved by using the programme PHASER [45] with the Hs HSD17B8 homotetramer (PDB id: 2PD6) as the starting model. The structure was initially refined using REFMAC5 (ref. 46 ) and at later stages twin refinement of Phenix.refine [44] was carried out. The estimated twin fraction is 0.3. The detection of twinning and the usage of the twin refinement option of ‘Phenix.refine’ greatly improved the resulting electron density maps as well as the refinement statistics. The structure was refined to a final R-free and R-work of 23.6% and 18.2%, respectively. Residues (94.9%) are in the favoured region of the Ramachandran plot, while 4.9% and 0.2% of the residues are in the allowed and outlier regions, respectively. The refinement statistics are presented in Table 1 . For Hs KAR crystals complexed with both NAD + and NADP + ( Hs KAR-NAD(P) + ), the X-ray diffraction data were collected at the Diamond Light Source, Oxford, UK, beamline I04 at a wavelength of 0.9795 Å using a PILATUS detector. The data were processed using the XDS package. The twin fraction for this crystal was much lower being <0.1. The Hs KAR-NAD + structure was used as the initial model to further build and refine the Hs KAR-NAD(P) + structure by the COOT and Phenix packages. The structure was refined to a final R-free and R-work of 23.6% and 20.3%, respectively. The distribution of residues in the Ramachandran plot is 93.3%, 3.5% and 0.1% in the favoured, allowed and outlier regions, respectively. A stereo image of a part of the 2 F o – F c electron density map of the Hs KAR-NAD + and Hs KAR-NAD(P) + structures is shown in Supplementary Fig. 6 . Structure validation and analysis The final structures were validated using Molprobity [47] . The α- and β-subunits of Hs KAR belong to the SDR superfamily. Of the four tetramers in the asymmetric unit, a single tetramer (chains A, B, C and D) was used for further analysis and comparison. The secondary structures assigned in Supplementary Fig. 1 follow previous nomenclature conventions [16] . The Hs KAR subunits were compared with homotetrameric KAR structures of the following species: (i) B. napus [13] (rape) (PDB id: 1EDU), (ii) E.coli [14] , [15] (PDB id: 1IO1 and 1Q7B) and (iii) Hs HSD17B8, the α-chain homotetramer (PDB id: 2PD6). The M. tuberculosis fabG4 (ref. 31 ) structure (PDB id: 3V1U) was used to study the ternary complex geometry. The structures were superimposed using the SSM option [48] in COOT [49] . The figures of the protein structures were drawn using PyMol (The PyMOL Molecular Graphics System, Version 1.5.0.3 Schrödinger, LLC). The web-based ClustalW2 programme was used to make the sequence alignment [50] . The sequence alignment figures were prepared using the program ESPRIPT [51] . Enzyme assays The catalytic activity of Hs KAR in the synthetic direction (the 3-ketoacyl-CoA reductase activity) was determined spectrophotometrically using a JASCO V660 spectrophotometer by monitoring the disappearance of NAD(P)H at 340 nm. Acetoacetyl-CoA was used as the substrate to assess the reductase activity. The reaction mixture contained 60 μM acetoacetyl-CoA and 125 μM NAD(P)H in 50 mM potassium phosphate buffer pH 7.4 with 100 μg ml −1 BSA in a final volume of 0.5 ml at 25 °C. The possible effect of Ca 2+ or Mg 2+ on the Hs KAR catalytic activity was verified [15] . These assays were therefore done also with additional 10 mM CaCl 2 or MgCl 2 . Although the use of CaCl 2 in assays resulted in the precipitation of buffer, MgCl 2 did not have any effect on the NAD(P)H-dependent activity. Hs CBR4 has previously been characterized to have in vitro quinone reductase activity [12] . Therefore, we also tested quinone reductase activity using 60 μM 9,10-PQ (Sigma-Aldrich, Steinheim, Germany) as the substrate in the reaction mixture (0.5 ml) containing also 125 μM NAD(P)H in 100 mM potassium phosphate buffer pH 7.5 with 50 μg ml −1 BSA. The reaction was initiated by adding 60 ng of Hs KAR and the disappearance of NAD(P)H at 340 nm was monitored. All the reported values for the enzymatic activity are the averages of at least three independent measurements and the reported errors are the s.d. of these measurements. Yeast spotting assay Yeast cells (BY4741 and BY4741 oar1 Δ mutant) were transformed with different combinations of plasmids by one-step transformation in stationary phase [52] . For each transformation, ~1 × 10 8 cells of stationary phase were collected from overnight cell culture by centrifugation and resuspended with 80 μl of yeast one-step transformation solution (100 mM lithium acetate, 33% PEG3350 and 0.28 mg ml −1 single-stranded DNA) and then mixed with 100 ng of plasmid DNA. The mixture was incubated at 45 °C for 45 min before plating. After transformation, the cells were plated on SC-Ura, SC-Leu, SC-Ura-Leu media containing 2% glucose. The colonies from plates were inoculated into appropriate selective liquid media and the cells were grown in a shaker at 30 °C until the OD 600 reached 8–10. The cells were then collected and spotted with a serial dilution on SC plates containing either 2% glucose or 3% glycerol as the sole carbon source and grown at 30 °C for 5–7 days. SPR studies Biacore T200 and the carboxymethyl-dextran-coated gold surface (CM5) sensor chip were used for the SPR measurements. Hs KAR at a concentration of 50 μg ml −1 in 10 mM sodium acetate buffer pH 5.0 was immobilized covalently by amine coupling on the CM5 chip, previously activated with 1-ethyl-3-(3-dimethylaminopropyl)carbodiimide hydrochloride and N-hydroxysuccinimide to ~9,500 RUs. The remaining reactive sites were blocked with ethanolamine. A reference cell was prepared in the same manner, except that Hs KAR was not injected. PBS buffer (1 × , pH 7.4) was used for all the measurements as well as for preparing the ligand solutions. The ligands, NAD + or NADP + , were passed over the chip containing Hs KAR at various concentrations ranging from 76 nM to 10 mM at a rate of 30 μl min −1 for 2 min. For NADH and NADPH, concentrations ranging from 76 nm to 40 mM were used. This was followed by a wash with PBS buffer pH 7.4 for 10–20 min to remove the bound ligands and regenerate the chip. This resulted in square pulses with fast association and dissociation rates ( Supplementary Fig. 4 ), and therefore the kinetics of ligand binding could not be studied. The K D values were calculated using either the two-site or the steady-state binding module of the Biacore T200 Evaluation software. For Hs KAR and αD42A- Hs KAR, sensograms of only up to 2.5 mM for NADP + and from 4.8 μM to 2.5 mM for NAD + were used for the calculation of K D . Moreover, for αD42A- Hs KAR sensogram from 40 mM NADPH and sensograms up to 2.4 μM NADH were not used for the determination of K D . The measurements were repeated at least three times and s.d. were calculated. Accession codes: The coordinates and the structure factor files for the crystal structure of the Hs KAR-NAD + and Hs KAR-NAD(P) + structures are deposited in the Protein Data Bank with the accession codes 4CQL and 4CQM , respectively. How to cite this article: Venkatesan, R. et al. Insights into mitochondrial fatty acid synthesis from the structure of heterotetrameric 3-ketoacyl-ACP reductase/3R-hydroxyacyl-CoA dehydrogenase. Nat. Commun. 5:4805 doi: 10.1038/ncomms5805 (2014).